SAPK pathways and p53 cooperatively regulate PLK4 activity and centrosome integrity under stress Polo-like kinase 4 is essential for centrosome duplication, but its hyperactivation causes supernumerary centrosomes. Here we report that polo-like kinase 4 is directly phosphorylated and activated by stress-activated protein kinase kinase kinases (SAPKKKs). Stress-induced polo-like kinase 4 activation promotes centrosome duplication, whereas stress-induced SAPK activation prevents centrosome duplication. In the early phase of stress response, the balance of these opposing signals prevents centrosome overduplication. However, in the late phase of stress response, p53 downregulates polo-like kinase 4 expression, thereby preventing sustained polo-like kinase 4 activity and centrosome amplification. If both p53 and the SAPKK MKK4 are simultaneously inactivated, as is frequently found in cancer cells, persistent polo-like kinase 4 activity combined with the lack of SAPK-mediated inhibition of centrosome duplication conspire to induce supernumerary centrosomes under stress. Indeed, tumour-derived MKK4 mutants induced centrosome amplification under genotoxic stress, but only in p53-negative cells. Thus, our results reveal a mechanism that preserves the numeral integrity of centrosomes, and an unexplored tumour-suppressive function of MKK4. Centrosomes, which consist of a pair of centrioles surrounded by an amorphous pericentriolar material, serve as the microtubule-organizing centres that are prerequisite for the formation of mitotic spindles in animal cells [1] , [2] . In order for cells to undergo normal bipolar cell division, the single interphase centrosome must duplicate precisely once before mitosis. Centrosome duplication is initiated at the G1/S transition and is completed during S phase. The rigorous control of centrosome numbers directs accurate chromosome segregation at cell division and is thus crucial for maintenance of the stability of genomes. The presence of more than two centrosomes (centrosome amplification) leads to the formation of multipolar mitotic spindles and consequently to chromosome-segregation errors [3] . Recent studies have shown that most cells with centrosome amplification can still undergo bipolar cell division, as multiple centrosomes cluster into two poles [4] , [5] . Centrosome amplification, however, significantly increases the frequency of lagging chromosomes during anaphase by causing erroneous, merotelic kinetochore-microtubule attachment, thereby promoting chromosome missegregation. Because chromosome missegregation results in both numerical (aneuploidy) and structural (translocations) abnormalities of chromosomes [6] , ablation of the numeral integrity of centrosomes induces chromosomal instability, and thus is considered to be a major cause of carcinogenesis and malignant progression. Indeed, centrosome amplification and the resulting chromosomal instability are common features of human cancers, and correlate with poor clinical outcomes [7] , [8] . Interestingly, centrosome number is often increased in cancer cells after various stress stimuli including DNA damage, oxidative stress and heat shock [9] , [10] , [11] , although the mechanism by which centrosome amplification arises after stress in cancer cells remains obscure. Polo-like kinase 4 (PLK4), a divergent member of the polo-like kinase family, is an evolutionarily conserved master regulator of centrosome duplication. PLK4 localizes to centrosomes and is essential for centriole biogenesis [12] . Depletion of PLK4 in cells leads to centrosome duplication arrest, whereas overexpression of PLK4 induces centrosome amplification by production of multiple procentrioles [13] , [14] . Previous reports have demonstrated that dysregulation (both hyperactivation and deactivation) of PLK4 predisposes cells to the development of cancer. PLK4 is expressed aberrantly (either over or underexpression) in human colorectal and liver cancers [15] , [16] . Mice heterozygous for PLK4 ( PLK4 +/− ) spontaneously develop liver and lung tumours, whereas PLK4 homozygous null mice are embryonic lethal [17] . Furthermore, overexpression of PLK4 promotes tumorigenesis in Drosophila [18] , [19] . Therefore, PLK4 activity must be adequately controlled to maintain centrosome integrity and to prevent carcinogenesis. During normal cell-cycle progression, the levels of PLK4 transcripts are low in G1, gradually increase through S and G2, and reach a maximum in mitosis [20] . Regulatory mechanisms of PLK4 activity, however, remain obscure. In particular, although PLK4 has been suggested to be involved in cellular stress responses [12] , [21] , it is unclear if (and how) PLK4 activity is regulated after stress, which frequently provokes centrosome amplification in cancer cells. In mammalian cells, stress stimuli elicit activation of specific intracellular signalling networks that regulate cell fates, ranging from survival to apoptosis. One of the major signalling systems that govern cellular stress responses is the p53 pathway. The tumour-suppressor p53 preserves genomic stability by triggering growth arrest or apoptosis after DNA damage and certain other cellular stresses [22] , [23] . In response to stress, p53 protein is gradually stabilized and accumulates in the nucleus, where it functions as a transcriptional regulator. Activated p53 interacts with sequence-specific DNA-binding sites and modulates, either positively or negatively, the expression of its target genes, thereby potentiating apoptosis. Another prominent event that responds rapidly to stress conditions is activation of the stress-activated p38 and JNK MAPK (SAPK) cascades [24] , [25] . The SAPK cascades consist of a three-tiered core of protein kinases, namely SAPKKK, SAPK kinase (SAPKK) and SAPK, and are activated by various stresses (for example, DNA damage, osmotic stress or oxidative stress) and by inflammatory cytokines (for example, tumour-necrosis factor-α (TNFα) or interleukin-1). Reflecting the presence of a wide range of cellular stresses, mammalian cells express more than a dozen SAPKKKs, such as MEKK1/2/3, MTK1 (also known as MEKK4), TAK1, ASK1, TAO1 and MLK1/2/3, each of which is activated in response to a distinct set of stimuli. Upon stress stimuli, these SAPKKKs activate a relatively limited number of their cognate SAPKKs (MKK3/4/6/7), which, in turn, activate SAPKs, thereby regulating reparative and/or apoptotic responses. Thus, both p53 and the SAPK pathways are critical for the dictation of cell-fate decisions in cells exposed to stress. Importantly, these signalling systems are frequently compromized in human cancers. In most cancers, p53 is inactivated, either by mutation or by other means including viral oncoproteins [26] . Furthermore, MKK4, the only SAPKK that can activate both p38 and JNK, is a target for inactivating mutations in various cancers, and is thus thought to be an important tumour suppressor [27] , [28] , [29] , although the precise mechanism by which MKK4 exerts its tumour-suppressor function remains elusive. Here we investigated how PLK4 is regulated by stress, and how such regulation relates to oncogenesis, with a particular emphasis on the interplay between PLK4, p53 and the SAPK pathways. Our data reveal a molecular mechanism that underlies centrosome amplification in cancer cells, in which the two tumour suppressors, p53 and MKK4, are frequently mutated. PLK4 binds to active forms of stress-responsive MAPKKKs To clarify the role, if any, of PLKs in cellular stress responses, we initially examined whether there is any functional cross-talk between PLKs and the SAPK pathways. In this examination, we found that PLK4 bound the kinase domain of the SAPKKK MTK1 (refs 30 , 31 ) ( Fig. 1a , lane 6). PLK4 did not bind to unactivated full-length MTK1, but it did so if GADD45β, a specific activator of MTK1 (ref. 32 ), was co-expressed ( Fig. 1a , lanes 3 and 4). Thus, only an active form of MTK1 bound to PLK4 through its kinase domain. Deletion analysis of PLK4 showed that two regions in PLK4, termed BD1 (261–491) and BD2 (762–970), could separately bind to MTK1 ( Fig. 1b ; Supplementary Fig. S1a,b ). PLK4 also preferentially bound to the active form of another SAPKKK, TAK1 ( Fig. 1c ). Interaction between endogenous PLK4 and TAK1 was detected by co-immunoprecipitation ( Fig. 1d ) from HeLa cells, synchronized in the G2/M phase, in which PLK4 was expressed at high levels (see Supplementary Fig. S1c ). Consistent with the transfection experiments, the binding of endogenous TAK1 to PLK4 was enhanced when cells were stimulated with osmotic stress (sorbitol), which activates TAK1 (refs 20 , 33 ) ( Fig. 1d ). 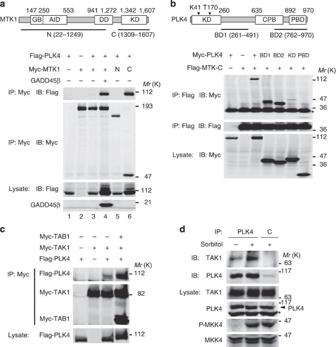Figure 1: Stress-responsive MAPKKKs bind PLK4. (a) Co-immunoprecipitation of Myc-MTK1 and Flag-PLK4. 293FT cells were transfected as indicated. Immunoprecipitated Myc-MTK1 was probed for co-precipitating Flag-PLK4. GB, GADD45-binding domain. AID, auto-inhibitory domain; C, C-terminal; DD, dimerization domain; KD, kinase domain; N, N terminal. (b) MTK1-binding domains in PLK4. CPB, cryptic Polo-box; PBD, Polo-box domain; *, IgG light chain. (c) PLK4 preferentially interacts with activated TAK1. 293FT cells were co-transfected with Myc-TAB1, Myc-TAK1 and Flag-PLK4. Immunoprecipitated Myc-TAK1 was probed for co-precipitating Flag-PLK4. (a–c) The levels of protein expression in cell lysates are also shown. (d) Association of endogenous PLK4 with TAK1 in HeLa cells treated with (+) or without (−) sorbitol. Phosphorylated MKK4 (P-MKK4) in the extracts was probed with an anti-phospho-MKK4 antibody (fifth). The expression level of MKK4 is also shown (bottom). C, control IgG; *, a non-specific band. Figure 1: Stress-responsive MAPKKKs bind PLK4. ( a ) Co-immunoprecipitation of Myc-MTK1 and Flag-PLK4. 293FT cells were transfected as indicated. Immunoprecipitated Myc-MTK1 was probed for co-precipitating Flag-PLK4. GB, GADD45-binding domain. AID, auto-inhibitory domain; C, C-terminal; DD, dimerization domain; KD, kinase domain; N, N terminal. ( b ) MTK1-binding domains in PLK4. CPB, cryptic Polo-box; PBD, Polo-box domain; *, IgG light chain. ( c ) PLK4 preferentially interacts with activated TAK1. 293FT cells were co-transfected with Myc-TAB1, Myc-TAK1 and Flag-PLK4. Immunoprecipitated Myc-TAK1 was probed for co-precipitating Flag-PLK4. ( a – c ) The levels of protein expression in cell lysates are also shown. ( d ) Association of endogenous PLK4 with TAK1 in HeLa cells treated with (+) or without (−) sorbitol. Phosphorylated MKK4 (P-MKK4) in the extracts was probed with an anti-phospho-MKK4 antibody (fifth). The expression level of MKK4 is also shown (bottom). C, control IgG; *, a non-specific band. Full size image SAPKKKs directly phosphorylate PLK4 at T170 Because PLK4 preferentially binds to active forms of SAPKKKs, we next investigated if SAPKKKs could regulate PLK4 activity by phosphorylation. For this purpose, we transfected HEK293 cells with Myc-PLK4 together with various activated SAPKKKs (either by expression of a constitutively active SAPKKK mutant or by co-expression of a SAPKKK and its specific activator) ( Fig. 2a ). Expression of active MTK1 (Flag-MTK1-C) elicited an upward band shift of co-expressed Myc-PLK4 in a western blot. Active forms of several other SAPKKKs (TAK1, MEKK1 or MLK3) could also induce a PLK4 band shift, whereas ASK1 or the mitogen-activated MAPKKK, c-Raf, could not. Phosphatase treatment showed that this PLK4 band shift was caused by phosphorylation ( Fig. 2b ). This band shift required the kinase activities of both MTK1 and PLK4, because it disappeared if kinase-dead mutants of MTK1(K/R) or PLK4(K/M or T/A) were used ( Fig. 2c , upper panel; Supplementary Fig. S2a ). These results raised the possibility that one of the kinases activated the other kinase. To determine if MTK1 affects PLK4 activity in vivo , Myc-PLK4 was immunoprecipitated from cell extracts, and its kinase activity was assessed in vitro using α-casein as an exogenous substrate ( Fig. 2c , lower panel). Co-expression of constitutively active Flag-MTK1-C, but not its kinase-dead mutant (K/R), strongly enhanced PLK4 activity. Thus, MTK1 kinase activity is required to activate PLK4 in vivo . The PLK4 band shift, however, likely results from autophosphorylation of activated PLK4. MTK1 did not activate PLK1, 2 or 3 ( Supplementary Fig. S2b ). The combined results suggest that various, if not all, SAPKKKs activate PLK4 in vivo . 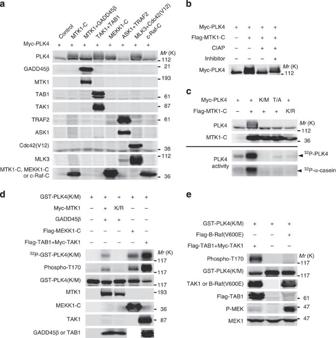Figure 2: Stress-responsive MAPKKKs phosphorylate and activate PLK4. (a) 293FT cells were transfected with Myc-PLK4, together with MAPKKKs and their activators as indicated. The induced band shift of Myc-PLK4 was analysed by immunoblotting. (b) The MTK1-induced PLK4 band shift is caused by phosphorylation. 293FT cells were co-transfected with Myc-PLK4 and constitutively active Flag-MTK1-C. Immunoprecipitated Myc-PLK4 was treated with calf-intestine alkaline phosphatase (CIAP) in the presence (+) or absence (−) of a phosphatase inhibitor mixture and was analysed by immunoblotting using an anti-Myc antibody. (c) MTK1 enhances PLK4 activity. The band shift (upper) andin vitrokinase activity (lower) of Myc-PLK4. α-Casein was used as an exogenous substrate for PLK4in vitro. K/M, PLK4(K41M); T/A, PLK4(T170A); K/R, MTK1(K1371R). (d,e) Stress-responsive MAPKKKs phosphorylate PLK4 at T170. Recombinant GST-PLK4(K41M) was incubated with immunoprecipitated MAPKKKsin vitro, and its phosphorylation status was monitored by32P incorporation (d) or by immunoblotting using an anti-phospho-PLK4(T170) antibody (d,e). Figure 2: Stress-responsive MAPKKKs phosphorylate and activate PLK4. ( a ) 293FT cells were transfected with Myc-PLK4, together with MAPKKKs and their activators as indicated. The induced band shift of Myc-PLK4 was analysed by immunoblotting. ( b ) The MTK1-induced PLK4 band shift is caused by phosphorylation. 293FT cells were co-transfected with Myc-PLK4 and constitutively active Flag-MTK1-C. Immunoprecipitated Myc-PLK4 was treated with calf-intestine alkaline phosphatase (CIAP) in the presence (+) or absence (−) of a phosphatase inhibitor mixture and was analysed by immunoblotting using an anti-Myc antibody. ( c ) MTK1 enhances PLK4 activity. The band shift (upper) and in vitro kinase activity (lower) of Myc-PLK4. α-Casein was used as an exogenous substrate for PLK4 in vitro . K/M, PLK4(K41M); T/A, PLK4(T170A); K/R, MTK1(K1371R). ( d , e ) Stress-responsive MAPKKKs phosphorylate PLK4 at T170. Recombinant GST-PLK4(K41M) was incubated with immunoprecipitated MAPKKKs in vitro , and its phosphorylation status was monitored by 32 P incorporation ( d ) or by immunoblotting using an anti-phospho-PLK4(T170) antibody ( d , e ). Full size image To determine how SAPKKKs activate PLK4, we employed in vitro kinase assays. For that purpose, we purified activated SAPKKKs (Myc-MTK1, Myc-TAK1 or Flag-MEKK1-C) from transfected 293FT cells and incubated them with kinase-dead GST-PLK4(K/M) that was expressed in bacteria. In vitro kinase assays using only these purified proteins showed that active MTK1, TAK1 and MEKK1, but not catalytically inactive MTK1(K/R), could directly phosphorylate GST-PLK4(K/M) ( Fig. 2d , top; Supplementary Fig. S2c,d ). To test if these kinases phosphorylate the essential activating phosphorylation site (T170) of PLK4 (ref. 20 ), we generated an antibody against phosphorylated T170 ( Supplementary Fig. S2e ). Immunoblot analyses using anti-phospho-T170 demonstrated that the SAPKKKs did phosphorylate T170 in vitro ( Fig. 2d , second row; Supplementary Fig. S2c,d ). Thus, these SAPKKKs can activate PLK4 by directly phosphorylating the activating phosphorylation site, T170. In contrast, constitutively active B-Raf(V600E) did not phosphorylate PLK4-T170 ( Fig. 2e ), which explains why Raf-family kinases could not activate PLK4 in vivo ( Fig. 2a ). Various stress stimuli activate PLK4 via SAPKKKs in vivo These in vitro results suggested that stresses that activate SAPKKKs would induce PLK4-T170 phosphorylation and PLK4 activation in vivo . To examine if osmotic stress activates PLK4, HEK293 cells transiently transfected with Myc-PLK4 were stimulated with 0.5 M sorbitol. Following sorbitol treatment, both PLK4-T170 phosphorylation ( Fig. 3a , top row) and the size of the PLK4 band shift ( Fig. 3a , middle row) gradually increased over ~60 min. Osmotic stress also enhanced PLK4 kinase activity ( Fig. 3b ). To exclude the possibility that activated PLK4 itself phosphorylates PLK4-T170, stress-induced T170 phosphorylation was examined in HEK293 cells stably expressing Myc-PLK4(K/M). The kinase-dead K/M mutation prevents any autophosphorylation event. Osmotic stress rapidly evoked PLK4-T170 phosphorylation even in these cells, concurrently with the activation of SAPKKKs, which was indicated by MKK4 phosphorylation ( Fig. 3c ; Supplementary Fig. S2f ). Other stresses (etoposide, ultraviolet or TNFα) also induced PLK4 phosphorylation ( Fig. 3d ; Supplementary Fig. S2g,h ). Thus, various stress stimuli activate PLK4 by inducing T170 phosphorylation in vivo . 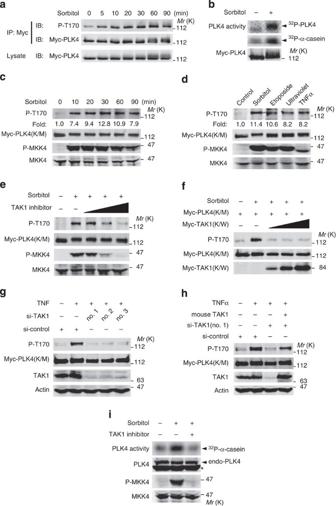Figure 3: Stress stimuli activate PLK4 via SAPKKKs. (a,b) 293FT cells transfected with Myc-PLK4 were stimulated with osmotic stress (0.5 M sorbitol). Immunoprecipitated Myc-PLK4 was analysed for T170 phosphorylation (a) or for its kinase activity in anin vitrokinase assay (b). (c,d) Immunoblotting of PLK4(T170) and MKK4 phosphorylation induced by various stress stimuli. HEK293 cells stably expressing Myc-PLK4(K41M) were stimulated with 0.5 M sorbitol for the indicated times (c), and with various stress stimuli as described in Methods (d). Phosphorylation states of PLK4(T170) and MKK4 were assessed by immunoblotting using anti-phospho-PLK4(T170) and anti-phospho-MKK4 antibodies, respectively (top and third). The same filters were reprobed with antibodies for total PLK4 and MKK4 (second and fourth). (e,f) PLK4(T170) phosphorylation was inhibited by the TAK1 inhibitor 5Z-7-oxozeaenol (e) or by dominant-negative TAK1(K63W) (f). (g,h) TAK1 knockdown suppresses PLK4(T170) phosphorylation induced by TNFα. HEK293 cells expressing Myc-PLK4(K/M) were transfected with a control siRNA or three distinct siRNAs specific for TAK1, and were stimulated with TNFα (50 ng ml−1for 20 min). Cell lysates were analysed by immunoblotting (g). Reintroduction of RNA interference-resistant mouse TAK1 restores T170 phosphorylation (h). (i) HeLa cells synchronized at the G2/M phase were stimulated with sorbitol in the presence or absence of the TAK1 inhibitor. Endogenous PLK4 was immunoprecipitated and its kinase activity was assessedin vitro(top). Phosphorylated MKK4 (P-MKK4) in the extracts was probed with an anti-phospho-MKK4 antibody (third). The expression levels of PLK4 and MKK4 in cell lysates are also shown (second and fourth). *, a non-specific band. Figure 3: Stress stimuli activate PLK4 via SAPKKKs. ( a , b ) 293FT cells transfected with Myc-PLK4 were stimulated with osmotic stress (0.5 M sorbitol). Immunoprecipitated Myc-PLK4 was analysed for T170 phosphorylation ( a ) or for its kinase activity in an in vitro kinase assay ( b ). ( c , d ) Immunoblotting of PLK4(T170) and MKK4 phosphorylation induced by various stress stimuli. HEK293 cells stably expressing Myc-PLK4(K41M) were stimulated with 0.5 M sorbitol for the indicated times ( c ), and with various stress stimuli as described in Methods ( d ). Phosphorylation states of PLK4(T170) and MKK4 were assessed by immunoblotting using anti-phospho-PLK4(T170) and anti-phospho-MKK4 antibodies, respectively (top and third). The same filters were reprobed with antibodies for total PLK4 and MKK4 (second and fourth). ( e , f ) PLK4(T170) phosphorylation was inhibited by the TAK1 inhibitor 5Z-7-oxozeaenol ( e ) or by dominant-negative TAK1(K63W) ( f ). ( g , h ) TAK1 knockdown suppresses PLK4(T170) phosphorylation induced by TNFα. HEK293 cells expressing Myc-PLK4(K/M) were transfected with a control siRNA or three distinct siRNAs specific for TAK1, and were stimulated with TNFα (50 ng ml −1 for 20 min). Cell lysates were analysed by immunoblotting ( g ). Reintroduction of RNA interference-resistant mouse TAK1 restores T170 phosphorylation ( h ). ( i ) HeLa cells synchronized at the G2/M phase were stimulated with sorbitol in the presence or absence of the TAK1 inhibitor. Endogenous PLK4 was immunoprecipitated and its kinase activity was assessed in vitro (top). Phosphorylated MKK4 (P-MKK4) in the extracts was probed with an anti-phospho-MKK4 antibody (third). The expression levels of PLK4 and MKK4 in cell lysates are also shown (second and fourth). *, a non-specific band. Full size image The p38 and JNK SAPK pathways are activated mainly through TAK1 in response to either osmotic stress or TNFα (refs 33 , 34 ). Therefore, we next investigated whether PLK4 phosphorylation induced by these stimuli is also mediated by TAK1. Indeed, inhibition of TAK1 activity either by use of a specific TAK1 inhibitor [35] , by co-transfection of a dominant-negative TAK1(K/W), or by TAK1-specific short interfering RNAs (siRNAs), abrogated PLK4 phosphorylation induced by osmotic stress or TNFα ( Fig. 3e–h for transfected PLK4; Fig. 3i for endogenous PLK4). In contrast, inhibition of the SAPK pathways at the level of SAPK using specific inhibitors of p38 and JNK, or at the level of SAPKK using dominant-negative MKK4(K/R), did not suppress PLK4-T170 phosphorylation ( Supplementary Fig. S3a,b ). We therefore concluded that TAK1 directly phosphorylated and activated PLK4 in response to osmotic stress or TNFα in vivo as well as in vitro . It is likely that different SAPKKKs phosphorylate and activate PLK4 in response to other stress stimuli. SAPKKK-mediated PLK4 activation occurs in the cytoplasm PLK4 shuttles between centrosomes and the cytoplasm [36] . To identify the cellular location where PLK4 binds to and is activated by SAPKKKs, we used an in situ proximity ligation assay (PLA), which can visualize specific protein–protein interactions within a cell [37] . HeLa cells were co-transfected with Flag-PLK4, Myc-MTK1 and GADD45β (an MTK1 activator), together with green fluorescent protein (GFP)-centrin as a centrosome marker. PLA signals arising from intermolecular interactions between active MTK1 and PLK4 were detected in the cytoplasm, but not in the centrosome ( Fig. 4a ). Similar results were also obtained for the interaction between TAK1 and PLK4 ( Fig. 4b ). Furthermore, subcellular fractionation indicated that endogenous PLK4 was present in both cytoplasmic and centrosomal fractions, whereas endogenous TAK1 was present only in the cytoplasm ( Fig. 4c ). Thus, SAPKKKs interact with and activate PLK4 primarily in the cytoplasm. It is, however, likely that stress-activated PLK4 is not limited to the cytoplasm but can be localized both in the cytoplasm and in the centrosome, because PLK4 rapidly shuttles between centrosomes and the cytoplasm [36] . 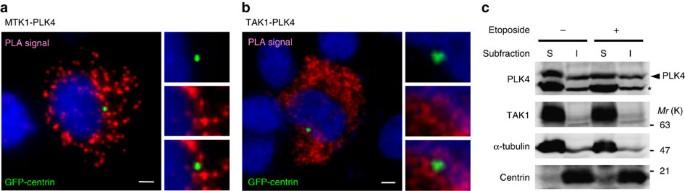Figure 4: SAPKKKs interact with PLK4 primarily in the cytoplasm. (a,b)In situvisualization of SAPKKK-PLK4 complexes using the PLA. HeLa cells were transfected with GFP-centrin, together with Myc-MTK1, GADD45β and Flag-PLK4 (a) or with HA-TAK1, Flag-TAB1 and Myc-PLK4 (b). The interaction between MTK1 and PLK4 (a) or between TAK1 and PLK4 (b) was visualized using PLA. Red, PLA signal; blue, 4′,6-diamidino-2-phenylindole; green, the centrosome marker GFP-centrin. Magnified images of the centrosome area are shown in the right insets. Scale bar, 5 μm. (c) Endogenous PLK4 is present in both soluble (cytoplasmic) and insoluble (centrosomal) fractions. G2/M-synchronized HeLa cells were lysed with PHEM buffer containing 1% Triton X-100 and separated into soluble (S) and insoluble (I) fractions. The expression level of PLK4 was assessed by immunoblotting. Endogenous TAK1, α-tubulin and centrin (a centrosome marker) were also probed as indicated. Figure 4: SAPKKKs interact with PLK4 primarily in the cytoplasm. ( a , b ) In situ visualization of SAPKKK-PLK4 complexes using the PLA. HeLa cells were transfected with GFP-centrin, together with Myc-MTK1, GADD45β and Flag-PLK4 ( a ) or with HA-TAK1, Flag-TAB1 and Myc-PLK4 ( b ). The interaction between MTK1 and PLK4 ( a ) or between TAK1 and PLK4 ( b ) was visualized using PLA. Red, PLA signal; blue, 4′,6-diamidino-2-phenylindole; green, the centrosome marker GFP-centrin. Magnified images of the centrosome area are shown in the right insets. Scale bar, 5 μm. ( c ) Endogenous PLK4 is present in both soluble (cytoplasmic) and insoluble (centrosomal) fractions. G2/M-synchronized HeLa cells were lysed with PHEM buffer containing 1% Triton X-100 and separated into soluble (S) and insoluble (I) fractions. The expression level of PLK4 was assessed by immunoblotting. Endogenous TAK1, α-tubulin and centrin (a centrosome marker) were also probed as indicated. Full size image PLK4 provides a survival signal that is downregulated by p53 To clarify the physiological relevance of stress-induced PLK4 activation, we first tested if PLK4 affects cellular stress responses. In this regard, a previous study has reported that PLK4 expression is transcriptionally repressed by the tumour-suppressor p53 (ref. 38 ). Indeed, following etoposide or ultraviolet treatment, the PLK4 protein gradually disappeared, accompanied by p53 accumulation, in p53-wt A549 cells, but the PLK4 protein persisted in the p53-null H1299 cells ( Fig. 5a ; Supplementary Fig. S4a ). Reintroduction of wild-type p53 into H1299 cells restored etoposide-induced suppression of PLK4 expression ( Fig. 5b ). These findings indicate that stress-induced PLK4 activity is gradually attenuated by the activation of p53. To investigate the role of PLK4 in the regulation of stress-induced apoptosis in the absence of any contribution from p53, PLK4 expression was knocked down by specific siRNAs in the p53-null H1299 cells ( Supplementary Fig. S4b ). PLK4 depletion by siRNA augmented etoposide-induced activation of caspase-9 (an initiator caspase), caspase-3 (an effector caspase) and the resulting proteolytic cleavage of PARP, which is a hallmark of apoptosis ( Fig. 5c ). Similar results were obtained using a distinct siRNA-targeting PLK4 ( Supplementary Fig. S4c ). Thus, increased kinase activity of PLK4 (mediated by SAPKKKs) suppressed apoptosis, whereas decreased expression of PLK4 (mediated by stress-induced p53) potentiated apoptosis. 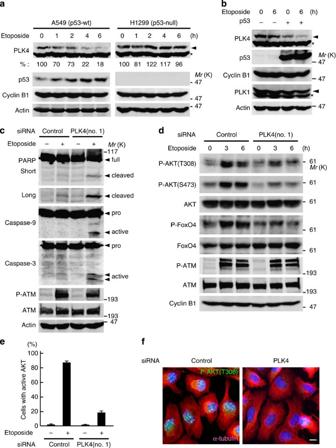Figure 5: p53 downregulates stress-induced PLK4 activity that suppresses apoptosis. (a) G2/M-synchronized A549 (wild-type p53) or H1299 (p53-null) cells were treated with etoposide (50 μM) for the indicated times. PLK4, p53, Cyclin B1 and actin (loading control) were probed by immunoblotting. *, a non-specific band. (b) p53-transfected H1299 cells were synchronized at the G2/M phase and stimulated with etoposide for 6 h. Cell lysates were immunoblotted with the indicated antibodies. *, a non-specific band. (c) PLK4 suppresses caspase-9-mediated apoptosis. H1299 cells transfected with PLK4 siRNA (no. 1) or control siRNA were treated with etoposide for 24 h. Cleavage of PARP, caspase-9 and caspase-3 was detected by immunoblotting. Short, short exposure; Long, long exposure. Levels of ATM phosphorylation at S1981 (P-ATM), which is induced by DNA damage, are comparable in cells transfected with control or PLK4 (no. 1) siRNA. (d–f) PLK4 mediates etoposide-induced activation of AKT. H1299 cells transfected with PLK4 siRNA (PLK4 (no. 1)) or control oligonucleotides were treated with etoposide (50 μM) for the indicated times (d) or for 3 h (e,f). Ind, phosphorylation levels of AKT at T308 and S473, FoxO4 at S197 and ATM at S1981 were detected by immunoblotting using appropriate phospho-specific antibodies (top, second, fourth and sixth rows). The expression levels of AKT, FoxO4, ATM and cyclin B1 in cell lysates are also shown (third, fifth, seventh and bottom). Ineandf, the indicated siRNA-transfected cells were treated with etoposide, fixed, and immuno-stained for phosphorylated AKT at T308 (green) and for α-tubulin (red). The percentage of cells stained with anti-phospho-AKT (T308) (active AKT) in the nucleus was determined (e). Error bars indicate s.e.m. (n=3), >200 cells counted per sample. Representative images were shown inf. As DNA was stained with 4′,6-diamidino-2-phenylindole (blue), P-AKT (green) in the nucleus appears as light blue. Scale bar, 10 μm. Figure 5: p53 downregulates stress-induced PLK4 activity that suppresses apoptosis. ( a ) G2/M-synchronized A549 (wild-type p53) or H1299 (p53-null) cells were treated with etoposide (50 μM) for the indicated times. PLK4, p53, Cyclin B1 and actin (loading control) were probed by immunoblotting. *, a non-specific band. ( b ) p53-transfected H1299 cells were synchronized at the G2/M phase and stimulated with etoposide for 6 h. Cell lysates were immunoblotted with the indicated antibodies. *, a non-specific band. ( c ) PLK4 suppresses caspase-9-mediated apoptosis. H1299 cells transfected with PLK4 siRNA (no. 1) or control siRNA were treated with etoposide for 24 h. Cleavage of PARP, caspase-9 and caspase-3 was detected by immunoblotting. Short, short exposure; Long, long exposure. Levels of ATM phosphorylation at S1981 (P-ATM), which is induced by DNA damage, are comparable in cells transfected with control or PLK4 (no. 1) siRNA. ( d – f ) PLK4 mediates etoposide-induced activation of AKT. H1299 cells transfected with PLK4 siRNA (PLK4 (no. 1)) or control oligonucleotides were treated with etoposide (50 μM) for the indicated times ( d ) or for 3 h ( e , f ). In d , phosphorylation levels of AKT at T308 and S473, FoxO4 at S197 and ATM at S1981 were detected by immunoblotting using appropriate phospho-specific antibodies (top, second, fourth and sixth rows). The expression levels of AKT, FoxO4, ATM and cyclin B1 in cell lysates are also shown (third, fifth, seventh and bottom). In e and f , the indicated siRNA-transfected cells were treated with etoposide, fixed, and immuno-stained for phosphorylated AKT at T308 (green) and for α-tubulin (red). The percentage of cells stained with anti-phospho-AKT (T308) (active AKT) in the nucleus was determined ( e ). Error bars indicate s.e.m. ( n =3), >200 cells counted per sample. Representative images were shown in f . As DNA was stained with 4′,6-diamidino-2-phenylindole (blue), P-AKT (green) in the nucleus appears as light blue. Scale bar, 10 μm. Full size image To gain insight into the molecular mechanism by which PLK4 inhibits apoptosis, we next investigated if PLK4 modulates functions of several key regulators of stress-induced apoptosis, such as the survival kinase AKT and Bcl-2 family proteins [39] , [40] . Depletion of PLK4 in H1299 cells by PLK4 siRNA markedly attenuated etoposide-induced activation of AKT, as demonstrated by its phosphorylation at T308 and S473 and by the phosphorylation state of an endogenous AKT substrate protein, FoxO4 ( Fig. 5d ). Immunofluorescence staining using an anti-phospho-AKT(T308) antibody further confirmed that depletion of PLK4 suppresses accumulation of active AKT in the nucleus following etoposide treatment ( Fig. 5e ). In contrast, PLK4 did not directly phosphorylate key members of tested Bcl-2 family proteins (Bax, Bak, Bcl-xL and Bcl-2) in vitro ( Supplementary Fig. S4d ). Thus, PLK4 protects cells from apoptosis by mediating stress-induced AKT activation. Based on the combined findings, we conclude that stress stimuli activate SAPKKKs, which then activate both pro-survival PLK4 and pro-apoptotic SAPK signalling [24] , [41] , [42] . At the same time, stress stimuli induce p53 that suppresses PLK4 expression. At first glance, these conflicting signals seem unproductive. However, the actual cell fate will be decided by the different timing of these signalling systems (see Fig. 8c, left panel). Stress-induced activation of PLK4 can take place only in the early phase of the stress response, because gradual activation of p53 will eventually eliminate PLK4 if the stress continues unabated. Therefore, we conclude that the PLK4 activation provides a time-limited survival signal in cells exposed to stress. SAPKs inhibit centrosome amplification Hyperactivation of PLK4 has been reported to drive centrosome overduplication that is marked by three or more centrosomes per cell [43] , [44] . Indeed, overexpression of Myc-PLK4 or hyper-stable Myc-PLK4-S285A/T289A (AA) [45] induced centrosome overduplication ( Fig. 6a ; Supplementary Fig. S5a ). Therefore, we next examined if SAPKKK-mediated PLK4 activation would also induce centrosome amplification. Unexpectedly, however, co-transfection of Myc-PLK4 with MTK1-C, which activates PLK4, was far less effective in evoking centrosome overduplication than Myc-PLK4 alone. One possible explanation of this result was that endogenous SAPKs (p38 and JNK) that were activated by MTK1-C might have inhibited centrosome overduplication. Indeed, co-expression of SAPKs together with MTK1-C and PLK4 further repressed centrosome overduplication ( Fig. 6a ). Moreover, expression of constitutively active p38 AS ( [46] ), even in the absence of co-transfected MTK1-C, suppressed PLK4-induced centrosome overduplication ( Fig. 6c ). Myc-p38 AS , however, inhibited neither PLK4-T170 phosphorylation nor PLK4 kinase activity ( Fig. 6d ; Supplementary Fig. S5c,d ), indicating that activated SAPKs block centrosome duplication without affecting PLK4. In theory, activated SAPKs could affect centrosome duplication indirectly by arresting the cell cycle. However, there was no substantial difference between the cell-cycle distribution of cells expressing PLK4 alone and those expressing both MTK1-C and PLK4 ( Supplementary Fig. S5b ). Moreover, Myc-p38 AS suppressed centrosome duplication even in aphidicolin-treated U2OS cells, in which centrosome duplication is uncoupled from the cell cycle [14] ( Fig. 6e ). Thus, p38 can inhibit centrosome duplication per se . 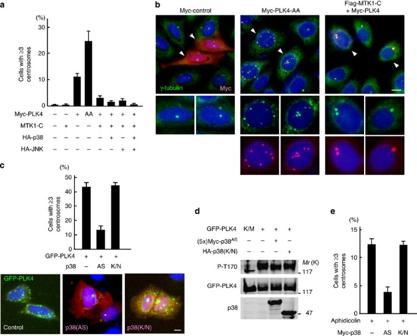Figure 6: SAPKs inhibit PLK4-induced centrosome overduplication. (a,b) HeLa cells were transfected as indicated. Two days after transfection, the percentage of transfected cells with ≥3 γ-tubulin dots (centrosome overduplication) was determined (a). Representative images of transfected cells (b). Magnified images of the centrosomes in cells indicated by the arrowheads are shown in the lower insets. Green, γ-tubulin; red, Myc; blue, 4′,6-diamidino-2-phenylindole. Scale bar, 10 μm. (c) HeLa cells were transfected with GFP-PLK4, and constitutively active p38ASor catalytically inactive p38(K53N) as indicated. Upper: percentage of GFP-positive cells with centrosome overduplication. Lower: green, GFP-PLK4; red, p38; blue, DNA. Scale bar, 5 μm. (d) p38 does not affect PLK4 activity. 293FT cells were transfected with constitutively active p38ASor catalytically inactive p38(K/N), together with kinase active or inactive (K41M) GFP-PLK4 as indicated. Immunoprecipitated GFP-PLK4 was probed for T170 phosphorylation. (e) p38 inhibits centrosome duplication induced by aphidicolin in U2OS cells. The percentage of transfected cells with ≥3 centrosomes was determined as ina. All data are the means of three independent experiments. Error bars indicate s.e.m., >200 cells counted per sample. Figure 6: SAPKs inhibit PLK4-induced centrosome overduplication. ( a , b ) HeLa cells were transfected as indicated. Two days after transfection, the percentage of transfected cells with ≥3 γ-tubulin dots (centrosome overduplication) was determined ( a ). Representative images of transfected cells ( b ). Magnified images of the centrosomes in cells indicated by the arrowheads are shown in the lower insets. Green, γ-tubulin; red, Myc; blue, 4′,6-diamidino-2-phenylindole. Scale bar, 10 μm. ( c ) HeLa cells were transfected with GFP-PLK4, and constitutively active p38 AS or catalytically inactive p38(K53N) as indicated. Upper: percentage of GFP-positive cells with centrosome overduplication. Lower: green, GFP-PLK4; red, p38; blue, DNA. Scale bar, 5 μm. ( d ) p38 does not affect PLK4 activity. 293FT cells were transfected with constitutively active p38 AS or catalytically inactive p38(K/N), together with kinase active or inactive (K41M) GFP-PLK4 as indicated. Immunoprecipitated GFP-PLK4 was probed for T170 phosphorylation. ( e ) p38 inhibits centrosome duplication induced by aphidicolin in U2OS cells. The percentage of transfected cells with ≥3 centrosomes was determined as in a . All data are the means of three independent experiments. Error bars indicate s.e.m., >200 cells counted per sample. Full size image To investigate if the converse is true, that is, if inhibition of SAPK activities would potentiate centrosome overduplication, we established mouse embryonic fibroblasts (MEFs) in which expression of a few or all of the SAPKKs (MKK3/4/6/7) were depleted. For this purpose, we used MKK3 −/− MKK6 −/− double-knockout MEFs (Δ3/6 MEFs) that are immortalized with the large T antigen [47] . The MKK4 and MKK7 genes in these cells were knocked down using specific short hairpin RNAs (shRNAs) to generate MEFs with the phenotype Δ3/6/4 or Δ3/6/4/7. As shown in Fig. 7a , stress-induced activation of SAPKs (p38 and JNK) was severely compromized in Δ3/6/4/7 MEFs, and was compromized to various degrees in Δ3/6 or Δ3/6/4 MEFs. As anticipated, the incidence of PLK4-induced centrosome overduplication in these MEFs showed an inverse correlation with the SAPK activities of the MEFs: lower SAPKK activities enhanced centrosome overduplication ( Fig. 7b ), whereas constitutively active SAPKKs (MKK3 EE and MKK6 DD ) or SAPK (p38 AS ) repressed centrosome overduplication ( Supplementary Fig. S5e ). Treatment with the genotoxic-stress agent etoposide, which activates SAPKs, evoked robust centrosome amplification, multipolar spindle formation and hyperploidy (>4N) in Δ3/6/4/7 MEFs, but not in wild-type cells ( Fig. 7c ; Supplementary Fig. S5f,g ). Thus, if stress stimuli activate PLK4 in the absence of SAPK activation, centrosome overduplication is induced, thereby leading to chromosomal instability and aneuploidy. Normally, however, simultaneous activation of PLK4 and SAPKs by stress stimuli prevents abnormal amplification of centrosomes under stress conditions. 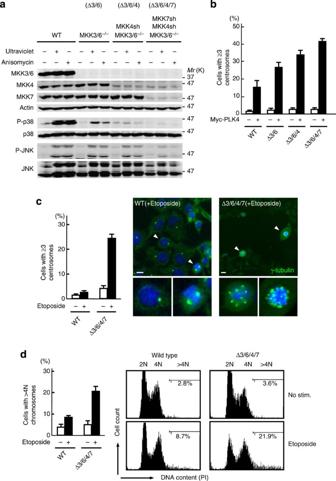Figure 7: Inhibition of SAPK activities potentiates stress-induced centrosome overduplication and aneuploidy. (a) Combined depletion of SAPKKs (MKK3, MKK6, MKK4 and MKK7) severely suppresses p38 and JNK activation in MEFs. Wild-type MEFs (WT), MKK3/6−/−MEFs (Δ3/6) and MKK3/6−/−MEFs stably expressing either an shRNA for MKK4 alone (Δ3/6/4) or together with an shRNA for MKK7 (Δ3/6/4/7) were stimulated with ultraviolet (80 J m−2followed by a 30-min incubation) or anisomycin (10 μg ml−1for 30 min). Expression levels of endogenous SAPKKs and the phosphorylation states of SAPKs (p38 and JNK) were analysed by immunoblotting. Actin served as a loading control. (b) WT or MEFs depleted of various SAPKKs (MKK3/6, MKK3/6/4 or MKK3/6/4/7) were transfected with Myc-PLK4 (+). Transfected cells with ≥3 centrosomes were counted as inFig. 6a. (c) WT or Δ3/6/4/7 MEFs were treated with etoposide (0.4 μM) for 8 h followed by recovery in drug-free medium for 2 days. Left: the numbers of centrosomes per cell were determined by γ-tubulin staining. Right: representative images of cells are shown. Green, γ-tubulin; blue, DNA. Scale bar, 10 μm. (d) Etoposide induces aneuploidy in Δ3/6/4/7 MEFs. WT and Δ3/6/4/7 MEFs were either left untreated (−) or were treated with etoposide (0.4 μM) for 8 h (+), followed by recovery in drug-free medium for 2 days. Cells were then fixed and stained with propidium iodide (PI). DNA content per cell was determined by fluorescence-activated cell sorting (FACS) analysis. The percentage of cells with >4 N chromosomes (left) and representative FACS results (right) are shown. (b–d) All data are the means of three independent experiments. Error bars indicate s.e.m., >200 cells counted per sample. Figure 7: Inhibition of SAPK activities potentiates stress-induced centrosome overduplication and aneuploidy. ( a ) Combined depletion of SAPKKs (MKK3, MKK6, MKK4 and MKK7) severely suppresses p38 and JNK activation in MEFs. Wild-type MEFs (WT), MKK3/6 −/− MEFs (Δ3/6) and MKK3/6 −/− MEFs stably expressing either an shRNA for MKK4 alone (Δ3/6/4) or together with an shRNA for MKK7 (Δ3/6/4/7) were stimulated with ultraviolet (80 J m −2 followed by a 30-min incubation) or anisomycin (10 μg ml −1 for 30 min). Expression levels of endogenous SAPKKs and the phosphorylation states of SAPKs (p38 and JNK) were analysed by immunoblotting. Actin served as a loading control. ( b ) WT or MEFs depleted of various SAPKKs (MKK3/6, MKK3/6/4 or MKK3/6/4/7) were transfected with Myc-PLK4 (+). Transfected cells with ≥3 centrosomes were counted as in Fig. 6a . ( c ) WT or Δ3/6/4/7 MEFs were treated with etoposide (0.4 μM) for 8 h followed by recovery in drug-free medium for 2 days. Left: the numbers of centrosomes per cell were determined by γ-tubulin staining. Right: representative images of cells are shown. Green, γ-tubulin; blue, DNA. Scale bar, 10 μm. ( d ) Etoposide induces aneuploidy in Δ3/6/4/7 MEFs. WT and Δ3/6/4/7 MEFs were either left untreated (−) or were treated with etoposide (0.4 μM) for 8 h (+), followed by recovery in drug-free medium for 2 days. Cells were then fixed and stained with propidium iodide (PI). DNA content per cell was determined by fluorescence-activated cell sorting (FACS) analysis. The percentage of cells with >4 N chromosomes (left) and representative FACS results (right) are shown. ( b – d ) All data are the means of three independent experiments. Error bars indicate s.e.m., >200 cells counted per sample. Full size image SAPKs and p53 cooperate to maintain centrosome integrity In the previous sections, we demonstrated that stress-activated SAPKs inhibit PLK4-mediated centrosome overduplication. Furthermore, stress-induced p53 downregulates PLK4 expression, thereby preventing its prolonged activation. Together, these findings imply that, under stress conditions, the numeral integrity of centrosomes is preserved by SAPKs and p53, which might act synergistically. Because both p53 and the MKK4 SAPKK are frequently impaired in human cancers [48] , we next tested a hypothesis that was based on the current findings, namely that combined inhibition of MKK4 and p53 might evoke centrosome amplification in cells exposed to genotoxic stress. To inactivate MKK4, we utilized two cancer-derived dominant-negative MKK4 mutants (N234I and S251N), which inhibit SAPK activation [49] . To inactivate p53 by proteasome-mediated degradation, we used the E6 gene of the human papilloma virus type 16 (HPV16) [50] . U2OS cells, in which both SAPK and p53 signalling are intact, were transfected with the dominant-negative MKK4 mutants and/or HPV16-E6, and were exposed to etoposide ( Fig. 8a ; Supplementary Fig. S6a ). Although the MKK4 mutants or HPV16-E6 individually had little effect on centrosome number, their combined expression significantly increased the incidence of supernumerary centrosomes. Similarly, depletion of MKK4 by siRNA in p53-null H1299 cells led to a higher incidence of supernumerary centrosomes compared with control H1299 cells, following etoposide treatment ( Supplementary Fig. S6b ). Thus, simultaneous inactivation of MKK4 and p53 increased the risk of centrosome amplification under stress conditions. 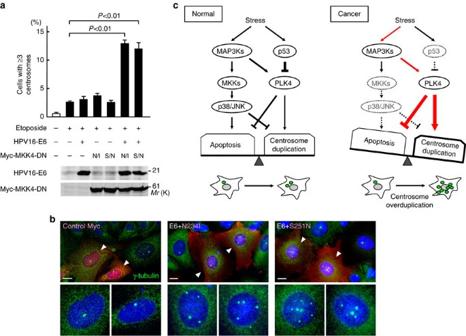Figure 8: p53 and SAPK signaling cooperate to maintain centrosome integrity under stress conditions. (a,b) U2OS cells were transfected with expression vectors for HPV16-E6 and/or cancer-derived Myc-MKK4 mutants (N234I or S251N), or with a control Myc-tag vector (−), as indicated. After 24 h, cells were treated with etoposide (0.8 μM) for 8 h, followed by 64 h recovery. The percentage of transfected cells with ≥3 centrosomes was determined as inFig. 6a. Error bars indicate s.e.m. (n=3), >200 cells counted per sample (a). Green, γ-tubulin; red, Myc; blue, DNA. Magnified images of the centrosomes in cells indicated by the arrowheads are shown in the lower insets. Scale bars, 10 μm (b). (c) A schematic model of a signalling network that regulate cell-fate decisions and centrosome integrity under stress conditions. In normal cells under stress (left), SAPKKKs concomitantly activate pro-survival PLK4 and pro-apoptotic SAPK signalling. PLK4 activation inhibits apoptotic cell death, particularly in the early phase of the stress response. If, however, the stress continues unabated, gradual activation of p53 leads to downregulation of PLK4 and promotes apoptosis. Furthermore, the numeral integrity of centrosomes is maintained under stress conditions by at least two distinct mechanisms. First, the activation of SAPKs inhibits PLK4-mediated centrosome overduplication. Second, p53-mediated downregulation of PLK4 prevents its prolonged activation. Thus, SAPK pathways and p53 cooperate to regulate cell-fate decisions and centrosome integrity under stress. In contrast, in cancer cells (right), when p53 and MKK4 are simultaneously inactivated by mutations, stress-induced PLK4 activation readily promotes centrosome overduplication, thereby inducing chromosomal instability and aneuploidy. See text for details. Figure 8: p53 and SAPK signaling cooperate to maintain centrosome integrity under stress conditions. ( a , b ) U2OS cells were transfected with expression vectors for HPV16-E6 and/or cancer-derived Myc-MKK4 mutants (N234I or S251N), or with a control Myc-tag vector (−), as indicated. After 24 h, cells were treated with etoposide (0.8 μM) for 8 h, followed by 64 h recovery. The percentage of transfected cells with ≥3 centrosomes was determined as in Fig. 6a . Error bars indicate s.e.m. ( n =3), >200 cells counted per sample ( a ). Green, γ-tubulin; red, Myc; blue, DNA. Magnified images of the centrosomes in cells indicated by the arrowheads are shown in the lower insets. Scale bars, 10 μm ( b ). ( c ) A schematic model of a signalling network that regulate cell-fate decisions and centrosome integrity under stress conditions. In normal cells under stress (left), SAPKKKs concomitantly activate pro-survival PLK4 and pro-apoptotic SAPK signalling. PLK4 activation inhibits apoptotic cell death, particularly in the early phase of the stress response. If, however, the stress continues unabated, gradual activation of p53 leads to downregulation of PLK4 and promotes apoptosis. Furthermore, the numeral integrity of centrosomes is maintained under stress conditions by at least two distinct mechanisms. First, the activation of SAPKs inhibits PLK4-mediated centrosome overduplication. Second, p53-mediated downregulation of PLK4 prevents its prolonged activation. Thus, SAPK pathways and p53 cooperate to regulate cell-fate decisions and centrosome integrity under stress. In contrast, in cancer cells (right), when p53 and MKK4 are simultaneously inactivated by mutations, stress-induced PLK4 activation readily promotes centrosome overduplication, thereby inducing chromosomal instability and aneuploidy. See text for details. Full size image In this study, we provide the first evidence for a direct functional link between the stress-responsive MAPK pathways and PLK4, a key regulator of centrosome number. In response to stress stimuli, PLK4 is directly phosphorylated and activated by SAPKKKs, thereby protecting cells from stress-induced apoptosis (see Fig. 8c ). Previous studies have shown that the abundance and activity of PLK4 are regulated by transcription, protein stability and phosphorylation [12] . In particular, PLK4 phosphorylation at T170 in the kinase activation loop is essential for the catalytic activity of PLK4 (ref. 20 ). The upstream kinases that are responsible for T170 phosphorylation, however, have not been identified. We found here that, under stress conditions, SAPKKKs directly phosphorylate PLK4 at T170. SAPKKK-mediated activation of PLK4 takes place primarily in the cytoplasm and specifically in response to stress. In contrast, a previous report showed that under normal exponential growth conditions, PLK4 activation occurs only at centrosomes [51] . In addition, activities of SAPKKKs are not significantly altered throughout the cell cycle in cells without stress, as monitored by MKK3/6 phosphorylation ( Supplementary Fig. S1c ). Therefore, SAPKKK-mediated PLK4 activation is specific for the regulation of cellular stress responses. The substrate specificity of SAPKKKs is relatively broad. For instance, several SAPKKKs phosphorylate inhibitor of nuclear factor κ-B kinase β (IKKβ) in addition to their cognate SAPKKs [24] . Here we showed that PLK4 is a novel substrate of several SAPKKKs. Thus, SAPKKKs not only activate the SAPK pathways but also initiate the PLK4 pathway within the same cell to trigger diverse, even opposing (survival or death), cellular responses. SAPKKK-mediated bifurcation of intracellular signalling might be critical for the dictation of cell-fate decisions depending on the type, strength and duration of stress stimuli. Indeed, we found that SAPKKK-mediated PLK4 activation suppressed apoptosis, particularly in the early phase of the stress response in cells with wild-type p53. Although the importance of PLK4 in the regulation of centrosome duplication has been well documented, less is known about the roles of PLK4 in other cellular processes. Accumulating evidence suggests that PLK4 also functions outside of the centrosome and is involved in controlling several essential cellular functions including cytokinesis and gene expression [16] , [21] . Furthermore, it should be noted that PLK4 −/− mice are embryonic lethal at E7.5 with a marked increase in apoptotic cells [17] , suggesting that PLK4 has a role in the regulation of apoptosis. We demonstrated here that under stress conditions, PLK4 serves as a pro-survival kinase and suppresses apoptotic cell death. Depletion of PLK4 by siRNAs significantly inhibited stress-induced AKT activation and thus augmented caspase-9-mediated apoptosis. AKT is activated not only by growth factors but also by a variety of stresses including DNA damage, although the molecular mechanism by which stress stimuli activate AKT is poorly understood [39] , [52] . Our results showed that PLK4 is a critical mediator of stress-induced AKT activation. Interestingly, PLK4 is transcriptionally repressed by p53 via the recruitment of histone deacetylase (HDAC) repressors [38] . Indeed, we showed that genotoxic stresses, such as etoposide treatment or ultraviolet irradiation, gradually downregulated PLK4 protein expression in a p53-dependent manner. Therefore, stress-induced, SAPKKK-mediated PLK4 activation provides a time-limited survival signal in p53 wild-type cells exposed to stress, and modulates the fate of cells in a manner that depends on the duration of the stress stimulus. Another even more important conclusion from our results is that the numeral integrity of centrosomes is preserved, under stress conditions, by both SAPKs and p53, which act synergistically ( Fig. 8c ). In normal cells under stress, SAPKs are rapidly activated and inhibit PLK4-mediated centrosome overduplication. Furthermore, when stress continues unabated, the tumour-suppressor p53 is gradually activated, and downregulates PLK4 to promote apoptosis and to reduce the risk of PLK4-induced centrosome amplification. Thus, SAPKs and p53 cooperate to maintain centrosome integrity under stress. The precise mechanism by which SAPKs inhibit centrosome overduplication remains to be elucidated. Our data, however, showed that the constitutively active SAPK, p38 AS , did not alter stress-induced PLK4 activity in vivo . Moreover, p38 AS suppressed aphidicolin-induced centrosome overduplication in U2OS cells. Thus, SAPKs directly prevent centrosome amplification by inhibiting centrosome duplication per se . Previous reports showed that a portion of activated p38 and JNK are localized in the centrosomes [53] , [54] , [55] , [56] . In addition, these SAPKs phosphorylate several molecules that can be localized in the centrosomes, such as the Cdc25 family of phosphatases, MK2, HSF1 and MNK1 (refs 55 , 57 , 58 ). Therefore, SAPKs might inhibit stress-induced centrosome amplification by phosphorylating these or other substrates in the centrosomes. Importantly, p53 and the SAPK pathways are frequently co-compromized in human cancer cells [26] , [28] . Furthermore, mutational inactivation of MKK4 has been shown to drive carcinogenesis (known as driver mutations). However, how MKK4 prevents carcinogenesis remains unclear [27] , [49] . Based on the present results, we propose the following mechanism for centrosome amplification in cancer cells (see Fig. 8c , right). When p53 is inactivated, cells fail to check the sustained PLK4 survival signal. Even under such conditions, activated SAPKs can still suppress centrosome overduplication. However, if an additional mutation occurs in the MKK4 gene, and both p53 and SAPK pathways are simultaneously impaired, stress-induced PLK4 activation readily promotes centrosome overduplication, thereby inducing chromosomal instability and aneuploidy. Centrosome amplification and chromosomal instability are hallmarks of cancer cells, and contribute to tumour aggressiveness [3] , [4] , [59] . Thus, our results provide a mechanistic insight into the molecular pathogenesis of centrosome alterations in human cancer, and highlight a novel tumour-suppressor role of MKK4. MKK4-mediated, robust activation of SAPKs protects cells from stress-induced centrosome amplification and consequent chromosomal instability in p53-negative cells. Therefore, the tumour-suppressive function of MKK4 is manifested particularly when p53 is also inactivated. Consistent with this notion, MKK4 mutations frequently coexist with p53 mutations in human cancer cells [48] . Given that PLK4 knockdown potentiated etoposide-induced apoptosis in p53-null cancer cells, PLK4 could be a potential therapeutic target for human cancer. Media and buffers Lysis buffer A contained 20 mM Tris-HCl (pH7.5), 1% Triton X-100, 0.5% deoxycholate, 10% glycerol, 137 mM NaCl, 2 mM EDTA, 54 mM β-glycerophosphate, 10 mM NaF, 2 mM sodium vanadate, 1 mM dithiothreitol, 1 mM phenylmethylsulphonyl fluoride, 10 μg ml −1 leupeptin and 10 μg ml −1 aprotinin. Lysis buffer B: Lysis buffer A without deoxycholate. Kinase buffer contained 25 mM Tris-HCl (pH 7.5), 25 mM MgCl 2 , 25 mM β-glycerophosphate, 0.5 mM sodium vanadate, 2 mM EGTA and 2 mM dithiothreitol. SDS–PAGE loading buffer consisted of 65 mM Tris-HCl (pH 6.8), 5% (vol/vol) 2-mercaptoethanol, 3% SDS, 0.1% bromophenol blue and 10% glycerol. Plasmids PLK4 was subcloned into pcDNA4Myc, pcDNA3Flag and pEGFP (Clontech) vectors using PCR. The mammalian expression plasmids for epitope-tagged MAPKKKs (pMyc-MTK1, HA-ASK1, Myc-TAK1, HA-TAK1, Flag-MEKK1-C, Flag-MLK3, Flag-BRaf(V600E), Flag-c-Raf-C and their derivatives], Myc-TAB1, GADD45β, Myc-GADD45β, Flag-TRAF2, GST-Cdc42(V12), HA-MKK3 EE , HA-MKK3(K/N), HA-MKK4, HA-MKK6 DD , HA-MKK6(K/N), Myc-p38 AS , HA-p38, HA-p38(K/N) and HA-JNK have been described [42] , [46] , [60] . To generate retroviral expression vectors, Myc-PLK4(K41M) or Myc-PLK4(K41M, T170A) were subcloned into pQCXIP (Invitrogen). The vector encoding HPV16-E6 (16E6SD-L151del) was from T. Kiyono [50] . Mutants were generated using PCR mutagenesis. Tissue culture HEK293, 293FT, HeLa, U2OS, A549 and H1299 cells were grown in DMEM and 10% FBS, and MEFs in high-glucose DMEM and 10% FBS. As indicated, cells were treated with sorbitol (0.5 M for 30 min), etoposide (50 μM for 3 h), ultraviolet (80 J m −2 followed by a 30-min incubation) or TNFα (50 ng ml −1 for 20 min). Transfections were performed using Effectene (Qiagen). The total amount of plasmid DNA was adjusted to 1 μg per plate with an empty vector. Co-immunoprecipitation assay Cell lysates were prepared in Lysis buffer B, precleared with protein G-sepharose beads at 4 °C for 1 h and incubated with an appropriate antibody immobilized on protein G-sepharose beads at 4 °C for 5 h. Immunoprecipitates were collected by centrifugation, washed four times with Lysis buffer B and subjected to SDS–PAGE. Immunoblotting analyses Immunoblotting analyses were carried out as described [60] . Digital images were captured using LAS-1000 Plus (Fujifilm). The following primary antibodies were used: mouse anti-Myc 9E10, anti-HA F7, anti-GST B-14, anti-GFP B-2, anti-MEK1 H-8 and anti-p53 DO-1 (Santa Cruz Biotechnology); mouse anti-Flag M2 (Sigma); rabbit anti-Myc, anti-p38, anti-JNK1, anti-ERK, anti-MKK4 and anti-MKK3/6 (Santa Cruz Biotechnology); rabbit anti-TAK1 (Sigma); goat anti-GADD45β (Santa Cruz Biotechnology); rabbit anti-phospho-MKK4, anti-phospho-MKK3/6, anti-phospho-MEK1/2, anti-phospho-p38, anti-phospho-JNK, anti-phospho-ERK, anti-phospho-MAPKAPK2, anti-phospho-c-Jun, anti-phospho-Aurora-A/B/C D13A11, anti-phospho-Akt(T308) C31E5E, anti-phospho-Akt(S473) D9E, anti-phospho-FoxO, anti-FoxO, anti-Akt, anti-PLK4 and anti-MKK7 (Cell Signaling); mouse anti-phospho-PLK1 2A3 (Abcam); anti-PLK1 35-206 (Zymed); anti-phospho-ATM 10H11.E12 (Cell Signaling); anti-Actin ACTN05 (Thermo); anti-Cyclin B1 V152 (MBL); anti-α-tubulin B-5-1-2 (Sigma); anti-Centrin 20H5 (Millipore); rabbit anti-PARP (Roche); anti-Caspase-3, anti-ATM D2E2 (Cell Signaling); and mouse anti-Caspase-9 5B4 (MBL). An affinity-purified anti-phospho-PLK4(T170) was made in-house. All antibodies were used at a dilution of 1:1,000, except anti-α-tubulin (diluted 1:5,000), anti-Cyclin B1 (diluted 1:10,000), anti-phospho-Akt(S473) (diluted 1:2,000) and anti-PARP (diluted 1:3,000). Proximity ligation assay HeLa cells grown on chamber slides were transfected with GFP-centrin (a centrosome marker), Flag-PLK4, Myc-MTK1 and GADD45β, or with GFP-centrin, Myc-PLK4, HA-TAK1 and Flag-TAB1. Thirty-six hours after transfection, PLA was performed using the Duolink in situ PLA kit (Olink Bioscience) according to the manufacturer’s protocol. The following primary antibodies were used at a dilution of 1:400: rabbit anti-Myc (Santa Cruz Biotechnology); mouse anti-Flag (Sigma); mouse anti-Myc (Santa Cruz Biotechnology); and rabbit anti-TAK1 (Sigma). Soluble/insoluble fractionation Soluble and insoluble fractions were prepared as described [51] . Briefly, HeLa cells synchronized in G2/M by thymidine-nocodazole treatment were washed with PBS and lysed in PHEM buffer (45 mM PIPES, 45 mM HEPES, 10 mM EGTA and 5 mM MgCl 2 , pH 6.9) containing 1% Triton X-100. Cell lysates were centrifuged at 300 g for 10 min at 4 °C. The supernatant (soluble fraction) was transferred to a new tube. The insoluble pellet (insoluble fraction) was washed with PHEM buffer and solubilized in a volume of SDS sample buffer by sonication on ice. Proteins in the soluble fraction were precipitated by adding 9 volumes of methanol, centrifuged at 4,000 g for 10 min at 4 °C, and the pellet was solubilized in the same volume of SDS loading buffer as that used for the insoluble fraction. In vitro kinase assay Immune-complex kinase assays were performed as described [32] . Briefly, cell extracts (in Lysis buffer A) were immunoprecipitated with the appropriate antibody for 4 h at 4 °C. Immune complexes were recovered with the aid of protein G-sepharose beads, washed twice with Lysis buffer B containing 500 mM NaCl, twice with Lysis buffer B and twice with kinase buffer. Immunoprecipitates were resuspended in 30 μl of kinase buffer containing 3 μg of GST-PLK4(K41M) (for MAPKKKs) or α-casein (for PLK4). The kinase reaction was initiated by the addition of [γ- 32 P] ATP, incubated for 30 min at 30 °C and terminated with SDS loading buffer. Incorporation of the radioactive phosphate group was visualized by autoradiography. GST-PLK4(K41M) was produced in E. coli using pGEX6P-1. Phosphatase assay Immunoprecipitated Myc-PLK4 was incubated with 55 U of calf-intestine alkaline phosphatase (Roche) in AP buffer (50 mM Tris-HCl pH 8.0, 100 mM NaCl and 10 mM MgCl 2 ) for 30 min at 25 °C. Phosphatase inhibitors were 25 mM β-glycerophosphate, 25 mM NaF and 2 mM sodium vanadate. Immunofluorescence staining Cells grown on glass coverslips were transfected with plasmids using Effectene and fixed with ice-cold methanol for 10 min. The cells were washed with PBS, permeabilized with 0.1% Triton X-100 for 5 min, incubated in the blocking solution BlockAce (Snow Brand) for 1 h, then incubated with the appropriate primary antibody (anti-γ-tubulin GTU-88 (Sigma); anti-Myc 9E10 (Santa Cruz Biotechnology); anti-Myc 9B11, anti-HA 6E2 (Cell Signaling); and anti-Centrin 20H5 (Millipore)) for 50 min in PBS containing 2% BSA. Following four PBS washes, cells were incubated for 30 min with the appropriate second antibody (Alexa Fluor 488-conjugated anti-mouse IgG1, Alexa Fluor 568-conjugated anti-mouse IgG or IgG2a, Cy2-conjugated anti-rabbit IgG or Dylight488-conjugated anti-rabbit IgG antibody). The coverslips were washed and mounted in FluorSave (Calbiochem). Fluorescence microscopic images were captured using a Nikon TE2000-E fluorescent microscope equipped with a Photometrics Cool-SNAP-HQ CCD camera, and the Universal Metamorph software (Molecular Devices) or Keyence BZ-9000 fluorescence microscope system. siRNA- or shRNA-mediated gene silencing Cells were transfected with siRNAs using Lipofectamine RNAiMAX (Invitrogen). The following siRNAs were used: si-TAK1 no. 1, 5′-AAAGCGUUUAUUGUAGAGCUUdTdT-3′; si-TAK1 no. 2, 5′-CCCGUGUGAACCAUCCUAAUAdTdT-3′; si-TAK1 no. 3, 5′-AACGGACAGCCAAGACGUAGAdTdT-3′; si-PLK4 no. 1, 5′-AAGGACUUGGUCUUACAACUAdTdT-3′; si-PLK4 no. 2, 5′-GGACCUUAUUCACCAGUUAdTdT-3′; si-MKK4 no. 1, 5′-AGGGUGUAUAGUGUUCACAAAdTdT-3′; si-MKK4 no. 2, 5′-UUGGACGAGGAGCUUAUGGUUdTdT-3′. The cells were subjected to various analyses 96 h (for si-TAK1), 72 h (for si-PLK4) or 48 h (for si-MKK4) after transfection. The shRNA expression vectors were constructed by inserting the following synthetic oligonucleotides into pSuper.retro vector: shRNA for mouse MKK4 (shMKK4), 5′-gatccccATGTCTACCTCGTTCGATAttcaagagaTATCGAACGAGGTAGACATttttta-3′; shRNA for mouse MKK7 (shMKK7), 5′-gatccccgTGAGATACTCGAGGTGGATttcaagagaATCCACCTCGAGTATCTCAttttta-3′. MKK3/6 −/− MEFs [47] were infected with retroviruses encoding shMKK4 and/or shMKK7, and the infected cells were selected using puromycin. Flow cytometry MEFs were treated with etoposide (0.4 μM) for 8 h followed by recovery in drug-free medium for 2 days. The cells were trypsinized, washed with PBS and fixed in 70% EtOH at −20 °C. Following a wash in PBS, the cells were stained with propidium iodide for 30 min and filtered through a cell-strainer. DNA content per cell was analysed by flow cytometry using Guava PCA (Millipore). Statistics The statistical significance of the difference between mean values was tested using Student’s t -test. Data are means±s.e.m. of at least three independent experiments. How to cite this article: Nakamura, T. et al . SAPK pathways and p53 cooperatively regulate PLK4 activity and centrosome integrity under stress. Nat. Commun. 4:1775 doi: 10.1038/ncomms2752 (2013).